Substrate-bound outward-open state of the betaine transporter BetP provides insights into Na+coupling The Na + -coupled betaine symporter BetP shares a highly conserved fold with other sequence unrelated secondary transporters, for example, with neurotransmitter symporters. Recently, we obtained atomic structures of BetP in distinct conformational states, which elucidated parts of its alternating-access mechanism. Here, we report a structure of BetP in a new outward-open state in complex with an anomalous scattering substrate, adding a fundamental piece to an unprecedented set of structural snapshots for a secondary transporter. In combination with molecular dynamics simulations these structural data highlight important features of the sequential formation of the substrate and sodium-binding sites, in which coordinating water molecules play a crucial role. We observe a strictly interdependent binding of betaine and sodium ions during the coupling process. All three sites undergo progressive reshaping and dehydration during the alternating-access cycle, with the most optimal coordination of all substrates found in the closed state. BetP, an osmotic-stress-regulated transporter from the betaine/choline/carnitine transporter family shares the conserved LeuT-like fold [1] of two inverted structural repeats of five transmembrane helices [2] , [3] ( Supplementary Movie ), whose pseudo-symmetry has been proposed as the mechanistic basis of the alternating-access mechanism of transport [4] . Various transporters from diverse sequence families share this highly conserved fold [5] , including other sodium-coupled transporters such as the hydantoin transporter Mhp1 [6] and a galactose transporter vSGLT [7] . Recently, several crystal structures of conformationally asymmetric BetP trimers have been reported [2] , which almost completed our view of the alternating-access cycle for BetP. Nevertheless, some fundamental questions were left unanswered. In particular, a substrate-bound outward-open state of BetP was missing and therefore the molecular understanding of the key events of substrate and co-substrate binding, and the subsequent transition to the closed state, was unclear. Recent structural work on BetP identified a functional important mutant (G153D) carrying an aspartate in the flexible stretch of transmembrane helix (TMH) 3, the first helix in the first repeat in LeuT-like fold transporters, which we denominate in the following as TMH1′. G153D is able to transport choline [8] ( Supplementary Movie ), exhibit an elevated apparent affinity for Na + and preferably crystallizes in an outward-facing state [2] . We have reported that crystallization of this mutant resulted in outward-facing open and outward-occluded apo states [2] . As most of the BetP structures exhibit only moderate resolution of ~3 Å, at which an unambiguous assignment of substrates to the electron density is hampered, here we co-crystallize BetP-G153D in the presence of a choline analogue containing arsenic instead of nitrogen, with which the substrate can be traced by arsenic anomalous scattering. These types of organo-arsenic compounds are natural constituents of many organisms, particularly from marine environments [9] . We show here that the slightly altered chemical nature of arseno-choline does not affect binding to BetP-G153D, although it leads to a reduction in K m compared with choline. Co-crystallization of BetP-G153D and arseno-choline result in crystals in which BetP adopts the missing substrate-bound outward-facing state, with arseno-choline bound to the central binding site and revealing the binding mode of choline in detail. Subsequently, we use the new outward-facing substrate-bound structure in molecular dynamics (MD) simulations to compare the detailed binding of substrate and sodium in outward-facing open (C e ), and outward-facing substrate-bound (C e S) states to that in the closed state (C c S) [2] , [10] . The results indicate that the two sodium ion-binding sites undergo major re-arrangements that affect their degree of hydration. Thus, the new C e S state represents a missing puzzle piece in what is now an unprecedented set of structural snapshots for a secondary transporter, that together emphasize the role of both sodium ions in shaping and finally closing the central substrate-binding site in accordance with the induced fit model. Binding and transport properties of arseno-choline Titration of BetP-G153D reconstituted in proteoliposomes with arseno-choline in the presence of 100 mM NaCl ( Fig. 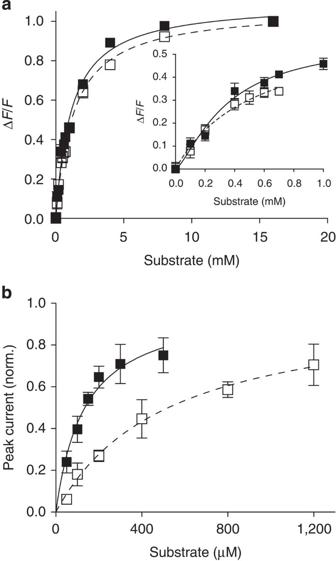Figure 1: Binding and transport properties of arseno-choline. Closed squares (choline), open squares (arseno-choline). (a) Tryptophan fluorescence-binding curve of choline and arseno-choline to BetP-G153D reconstituted in proteoliposomes. Each point shows the average for eight individual measurements. The error bars represent s.d. (b) Normalized peak currents of sodium-coupled transport of choline and arseno-choline to BetP-G153D. The graphs show average values from three individual recordings and the corresponding s.d. 1a ) revealed a similar binding affinity to that of choline ( Supplementary Table 1 ). The arseno-choline-binding isotherm reveals biphasic-binding behaviour and positive cooperativity ( n Hill =1.69±0.08), similar to the binding behaviour of choline. Arsenic sustains two additional electron shells relative to nitrogen. Thus, the coordination of the trimethylarsonium group may differ slightly from that of trimethylammonium, which involves cation-π interactions with tryptophan residues in the substrate-binding site [2] . However, the substrate hydroxyl group appears to interact with the carboxylic side chain [8] of Asp153, which may suffice to compensate for any differences owing to the As atom so that the binding affinity is comparable to that of choline. To demonstrate transport of arseno-choline, solid-supported membrane (SSM)-based electrophysiology was performed with proteoliposomes of reconstituted [10] BetP-G153D. A transient current corresponding to transmembrane charge displacement was detected after activation with arseno-choline, showing that this compound can be transported ( Fig. 1b ). The peak maximum current plotted as a function of substrate concentration showed a fourfold increase in K m for arseno-choline ( K m =523±70 μM) compared with that of choline ( K m =135±28 μM) ( Fig. 1b ; Supplementary Table 1 ), suggesting some effect of the larger trimethylarsonium group on the transport kinetics of this substrate. Nevertheless, our thermodynamic and kinetic studies of arseno-choline indicate that the arseno derivative can be considered a suitable substrate analogue. Therefore, we included this compound in co-crystallization trials, allowing us to trace binding to BetP-G153D using arsenic anomalous scattering. Figure 1: Binding and transport properties of arseno-choline. Closed squares (choline), open squares (arseno-choline). ( a ) Tryptophan fluorescence-binding curve of choline and arseno-choline to BetP-G153D reconstituted in proteoliposomes. Each point shows the average for eight individual measurements. The error bars represent s.d. ( b ) Normalized peak currents of sodium-coupled transport of choline and arseno-choline to BetP-G153D. The graphs show average values from three individual recordings and the corresponding s.d. 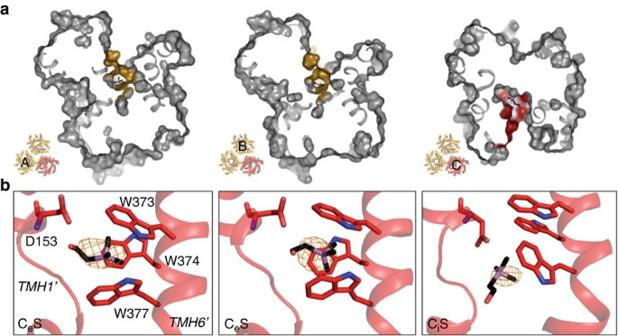Figure 2: Conformational states and arseno-choline binding observed in BetP-G153D. (a) Surface representation showing the periplasmic cavity. Chains A and B are in substrate-bound outward-open state (CeS), while chain C is in substrate-bound inward-open conformation (CiS). (b) Central binding sites of chains A, B and C, respectively. Arseno-choline is shown in black, red and purple sticks. Anomalous difference Fourier maps are shown at 4.0σ, 7.0σ and 4.0σ levels for substrates in chain A, B and C, respectively. Full size image An arseno-choline-bound outward-open state (C e S) Co-crystallization of BetP-G153D with arseno-choline yielded crystals diffracting to 2.95 Å resolution ( Supplementary Table 2 ). As observed previously for this mutant, the crystal structure reveals an asymmetric trimer [2] , although unlike the earlier crystal structure, chain A and B adopt an arseno-choline-bound outward-open conformation (C e S), and chain C an arseno-choline-bound inward-open conformation (C i S) ( Fig. 2a ). The previous crystal structure of BetP-G153D contained substrate-free outward-occluded (C eoc ) and outward-open states (C e ) [2] . The appearance of the outward-facing state found exclusively in crystals of this mutant was attributed to the sixfold higher apparent affinity for sodium, which presumably stabilizes this conformation by occupation of the Na2 site [11] , [12] . The new C e S state that we report here is also not frequently observed in the LeuT-like fold family. Indeed, only structures of the amino-acid antiporter AdiC have been observed in a similar C e S state [13] , while for LeuT only the competitive inhibitor-bound outward-open state [14] has been reported ( Supplementary Fig. 1 ). Figure 2: Conformational states and arseno-choline binding observed in BetP-G153D. ( a ) Surface representation showing the periplasmic cavity. Chains A and B are in substrate-bound outward-open state (C e S), while chain C is in substrate-bound inward-open conformation (C i S). ( b ) Central binding sites of chains A, B and C, respectively. Arseno-choline is shown in black, red and purple sticks. Anomalous difference Fourier maps are shown at 4.0σ, 7.0σ and 4.0σ levels for substrates in chain A, B and C, respectively. Full size image In this study, we used an oversaturating concentration of arseno-choline (approximately eightfold above K d ~1 mM), which appears to preferentially populate the C e S state, presumably owing to the distinct binding and transport characteristics of this substrate. Thus, the structures of protomers A and B, which we assign to the C e S state, contain a fully open central cavity that renders the central substrate and co-substrate-binding sites sterically accessible from the periplasm, whereas a ~18-Å-thick protein density occludes these sites from the cytoplasm ( Fig. 2a ). By contrast, in protomer C the central binding site is fully accessible to the cytoplasm, and is therefore assigned to the C i S state ( Fig. 2a ). An anomalous difference Fourier map revealed prominent peaks in the central binding sites of chains A, B and C ( Fig. 2b ). These could be observed when using a contour level of up to 6.1σ for chain A, 11.8σ for chain B and 5.2σ for chain C. No additional arsenic anomalous peaks were observed at comparable contour levels besides the ones in the central binding sites, indicating that, at least in these conformations of G153D, other high affinity arseno-choline-binding sites could not be discerned. Similar to what was observed for the C c S state [1] , the binding site in the C e S state is formed by three tryptophan residues from TMH6′ arranged as in a prism (Trp-prism); Trp373, Trp374 and Trp377 coordinate the trimethylarsonium group of the substrate, while the carboxyl group of Asp153 and the backbone amide of Gly151 appear to hydrogen bond with the hydroxyl group of arseno-choline ( Fig. 2b ). During multiple 200-ns-timescale MD simulations of C e S monomers of BetP-G153D embedded in a hydrated bilayer of POPG lipids, these hydrogen bonds are readily formed, and the same overall coordination is maintained throughout ( Fig. 3 ), providing confidence in the choice of arseno-choline as a substrate analogue. A similar interaction between a side-chain carboxyl group and the hydroxyl group of choline has been observed in other choline-binding proteins, including: the substrate-binding protein ChoX of the ABC transporter ChoXWU from Escherichia coli [15] ; the major autolysin (C-Lyta) from Streptococcus pneumoniae [16] ; and the choline-binding protein OpuBC from Bacillus subtilis [17] . This similarity indicates parallels in the binding modes of choline in membrane and soluble proteins. 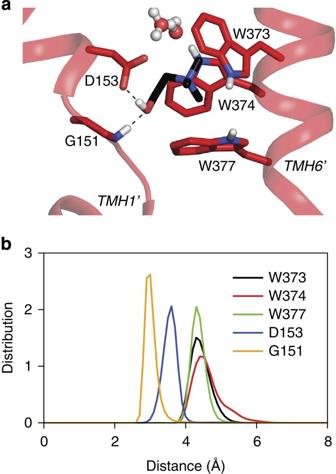Figure 3: CeS state coordination of choline in the S1-binding site of BetP-G153D. (a) Typical coordination of choline (black sticks) during the MD simulations by TMH1′ and TMH6′ (cartoon helices). Key residues (sticks) and water molecules (ball-and-stick) are shown. Non-covalent interactions are shown as dashed lines. (b) Distances were measured between the N atom of choline and the center of mass of the side chains in the tryptophan box (W377, W374 and W377), or between the hydroxyl oxygen of choline and the N backbone atom of G151 or the closest carboxyl oxygen atom of D153. The distribution was calculated over three trajectories, each 200 ns long. Figure 3: C e S state coordination of choline in the S1-binding site of BetP-G153D. ( a ) Typical coordination of choline (black sticks) during the MD simulations by TMH1′ and TMH6′ (cartoon helices). Key residues (sticks) and water molecules (ball-and-stick) are shown. Non-covalent interactions are shown as dashed lines. ( b ) Distances were measured between the N atom of choline and the center of mass of the side chains in the tryptophan box (W377, W374 and W377), or between the hydroxyl oxygen of choline and the N backbone atom of G151 or the closest carboxyl oxygen atom of D153. The distribution was calculated over three trajectories, each 200 ns long. Full size image This position of the arseno-choline in the C e S conformations differs from that in the C i S state, where the trimethylarsonium group is displaced from the Trp-prism ( Fig. 2b , right). The latter is similar to what was observed for choline as well as for betaine in the C i S state of a previously reported structure [8] . Analysis of the B-factors ( Supplementary Fig. 2 ) and root mean-squared fluctuations ( Supplementary Fig. 3 ) of the substrate-binding site residues in the C e S state suggest that the unwound segment of TMH1′ and perhaps also residues Trp373 and Trp377 of TMH6′ that form the Trp-prism, increase their conformational rigidity upon substrate binding, as compared with the C e state of BetP ( Supplementary Fig. 2 ). Although such a comparison of B-factors should be considered with caution because the structures differ, a similar trend is observed on comparison of the related states for AdiC and LeuT ( Supplementary Fig. 2 ) for the unwound segments of TMH1′ and for TMH6′, in which B-factors are reduced for the residues involved in substrate or competitive inhibitor binding, respectively [13] , [14] . Such entropic changes could conceivably facilitate the conformational changes between outward- and inward-facing states, imposing a dependence of the transition on substrate and co-substrate binding. The Na2 sodium-binding site in the C e S state NaCl titration of BetP-G153D reconstituted in proteoliposomes revealed positive cooperativity ( n Hill =1.9±0.2) [2] , similar to that observed for wild-type (WT) BetP [2] . This cooperativity suggests that the mutant retains the two-Na + binding stoichiometry of WT BetP [10] . Recently, two sodium-binding sites in BetP were localized and functionally validated based on a crystal structure of the C c S state, symmetry considerations and molecular simulations [10] . The Na2 site is highly conserved among symporters of the LeuT-like superfamily [18] , and a positive peak in the Fo-Fc electron-density map was observed at this site in the earlier BetP C c S structure [2] . We detected an equivalent peak in the Fo-Fc electron-density map at the Na2 site in the new C e S state structures ( Fig. 4a ), suggesting that sodium is bound to the Na2 site in the substrate-bound outward-open (C e S) conformation. This proposal is supported by the fact that a Na + was stably coordinated at this Na2 site during multiple 200-ns-long MD simulations of the BetP-G153D C e S state ( Fig. 4b–e ). 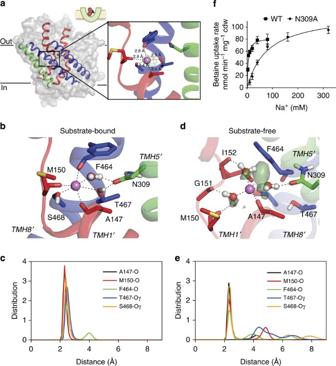Figure 4: The Na2-binding site in outward-open states of BetP-G153D. (a) The CeS state structure (protomer B) in side view with Na2 and adjacent central substrate-binding site in stick representation, coordinating Na+(violet sphere) and arseno-choline (black, red and purple sticks), respectively. The inset shows the coordination of a Na+ion (violet sphere) in the Na2 site. TheFo−Fcelectron density map is shown in green at a level of 3.0σ. (b–e) The Na2 site in simulations of the substrate-bound CeS (b,c) and substrate-free Ce(d,e) states: (b,d) Example configurations in simulations of the CeS state (b) and the Cestate (d). Proteins and ions are presented as in (a), waters are shown as balls-and-sticks and water densities are shown as green surfaces. (c,e) Distance between Na+ion and Na2-site oxygen atoms during three molecular dynamics simulations of the substrate-bound CeS state (c), each 200 ns long, and the substrate-free Cestate (e), each 100 ns long. (f) Betaine uptake rates in nmol min−1mg−1cell dry weight (cdw) were measured as a function of the external sodium concentration inE. coliMKH13 cells expressing BetP WT or the mutant N309A. Each point shows the average of at least three independent experiments. Error bars represent s.d. Figure 4: The Na2-binding site in outward-open states of BetP-G153D. ( a ) The C e S state structure (protomer B) in side view with Na2 and adjacent central substrate-binding site in stick representation, coordinating Na + (violet sphere) and arseno-choline (black, red and purple sticks), respectively. The inset shows the coordination of a Na + ion (violet sphere) in the Na2 site. The F o −F c electron density map is shown in green at a level of 3.0σ. ( b – e ) The Na2 site in simulations of the substrate-bound C e S ( b , c ) and substrate-free C e ( d , e ) states: ( b , d ) Example configurations in simulations of the C e S state ( b ) and the C e state ( d ). Proteins and ions are presented as in ( a ), waters are shown as balls-and-sticks and water densities are shown as green surfaces. ( c,e ) Distance between Na + ion and Na2-site oxygen atoms during three molecular dynamics simulations of the substrate-bound C e S state ( c ), each 200 ns long, and the substrate-free C e state ( e ), each 100 ns long. ( f ) Betaine uptake rates in nmol min −1 mg −1 cell dry weight (cdw) were measured as a function of the external sodium concentration in E. coli MKH13 cells expressing BetP WT or the mutant N309A. Each point shows the average of at least three independent experiments. Error bars represent s.d. Full size image We note that the Na2 site coordination in this outward-open state differs slightly from that in structures of the closed C c S state [2] . For example, there are occasional fluctuations in the coordination by the F464 backbone carbonyl of C e S ( Fig. 4e ). Interestingly, the coordination of the Na2 site involves Asn309 from the gating helix TMH5′ ( Fig. 4c,d ). Asn309 is at the equivalent position of the key cation-substituting group Arg262 in a sodium-independent antiporter, CaiT [19] , and is one turn above the position equivalent to Asp189 in vSGLT, which is thought to interact with the Na2 ion in that transporter [20] , [21] . We tested the importance of this residue for BetP by replacing Asn309 with alanine. Uptake assays in E. coli MKH13 cells reveal that this substitution increases the apparent K m of BetP for sodium ~20-fold ( Fig. 4f ; Table 1 ) compared with that of BetP WT, confirming the predicted role of Asn309 in the sodium dependence of substrate transport, and suggesting that the interaction observed in the C e S simulations is physiologically important. Table 1 Kinetic parameters for apparent sodium affinity measured from betaine uptake of WT BetP and N309A mutant. Full size table Unlike the aforementioned C e S- and C c S-state structures of BetP, no positive peak was detected at the Na2 site in the substrate-free outward-facing state [2] (C e ). This lack of a positive peak is consistent with the observed distortion of the binding site in the C e structure ( Table 2 ) owing to a number of subtle changes in the structure. These changes are: a ~2-Å displacement and unwinding of the middle of TMH8′ near Phe464; a ~2-Å vertical translation of the cytoplasmic half of TMH3′ towards the site; as well as a shift in the unwound segment of TMH3′ away from the site. As a result, Thr467 and Met150 appear no longer close enough to coordinate the ion in the C e state compared with the C e S state ( Fig. 5a,b ). Indeed, during simulations of C e structures, an ion in the Na2 region was unable to interact with all ligands simultaneously, and mainly interacted with Ala147, Phe464 and Ser468 ( Fig. 4d,e ). Nevertheless, the ion did not escape from the C e -Na2 site during these simulations, unlike ions placed in the Na2 site of inward-facing (C i ) states of other transporters such as vSGLT [22] and Mhp1 [6] , where all contributing oxygen atoms are >2 Å further apart than in the C e state ( Table 2 ), so that the site is effectively abolished. Instead, in simulations of C e , the Na + ion maintained coordination by one or other backbone oxygen of TMH3′ ( Fig. 4d ), as well as an average of 2.0±0.8 water molecules within 3 Å of the ion ( Fig. 3e ). The high degree of hydration of the C e -Na2 site is consistent with the lack of a clear peak. This behaviour is distinct from ions at Na2 in the inward C i S or closed C c S states, where the site is fully disrupted (and solvent accessible) or fully formed (and completely inaccessible), respectively [10] ( Table 2 ). Table 2 Na + -binding site integrity in different states of BetP measured as the distance between coordinating groups in X-ray crystallographic structures and during molecular dynamics simulations thereof. 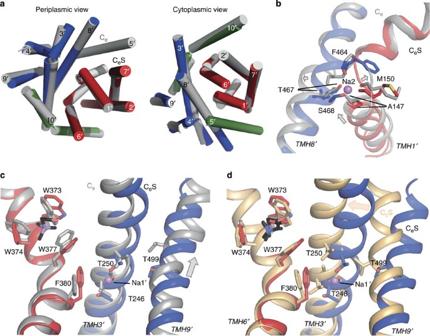Figure 5: Ion-binding sites in outward-facing and closed states of BetP. Structures and ion-binding sites in CeS (colours), Ce(grey) and CcS (tan) states of BetP and BetP-G153D are compared. Sodium ions (violet spheres), and substrate (black sticks) are shown. Changes from the CeS state to the compared state are indicated using arrows. (a–c) Comparisons of substrate-free Ce(PDB entry 4DOJ chain B, grey) and substrate-bound CeS states (colours), showing the effect of substrate binding on the outward-open states on: (a) the overall structure, with helices shown as cylinders; (b) the Na2-binding site, showing protein (ribbons), binding site residues (sticks) and Na2 ion from the CeS structure (sphere). (c) The substrate site (S1) and Na1′ site, with protein shown as ribbons, and with substrate (black) and binding-site residues as sticks. The location of the Na1′ ion is taken from the CeS simulations. (d) Comparison of Na1′ and substrate (S1)-binding site regions in the substrate-bound outward-open (CeS, colours) and the substrate-bound closed (CcS; PDB entry 4AIN chain B, tan) states. The Na1′ ion location is taken from the CeS simulations. Full size table Figure 5: Ion-binding sites in outward-facing and closed states of BetP. Structures and ion-binding sites in C e S (colours), C e (grey) and C c S (tan) states of BetP and BetP-G153D are compared. Sodium ions (violet spheres), and substrate (black sticks) are shown. Changes from the C e S state to the compared state are indicated using arrows. ( a – c ) Comparisons of substrate-free C e (PDB entry 4DOJ chain B, grey) and substrate-bound C e S states (colours), showing the effect of substrate binding on the outward-open states on: ( a ) the overall structure, with helices shown as cylinders; ( b ) the Na2-binding site, showing protein (ribbons), binding site residues (sticks) and Na2 ion from the C e S structure (sphere). ( c ) The substrate site (S1) and Na1′ site, with protein shown as ribbons, and with substrate (black) and binding-site residues as sticks. The location of the Na1′ ion is taken from the C e S simulations. ( d ) Comparison of Na1′ and substrate (S1)-binding site regions in the substrate-bound outward-open (C e S, colours) and the substrate-bound closed (C c S; PDB entry 4AIN chain B, tan) states. The Na1′ ion location is taken from the C e S simulations. Full size image In summary, these results suggest that the coordination of the Na2 site becomes progressively optimized as the protein transitions from the C e through the C e S to the C c S states, where it adopts the most optimal coordination. The Na1′ sodium-binding site in the C e S and C e states The position of the second sodium-binding site was recently proposed based on the structural symmetry between repeats [10] , and the proposal for this so-called Na1′ site (which is distinct from the Na1 site in LeuT) was validated using biophysical assays and molecular simulations [10] . That study indicated a sodium ion at this position in the C c S state would be coordinated by the hydroxyl groups of Thr246 and Thr250 from TMH3′, by a water molecule that hydrogen bonds to Thr499 from TMH9′, and potentially by a cation-π interaction to the aromatic ring of Phe380 from TMH6′. Although no positive peak for a Na1′ sodium ion was observed in the Fo-Fc electron-density map of the outward-facing C e S state ( Fig. 6a ), molecular simulations of this C e S state indicated that an ion at the Na1′ site interacts with the two Thr residues in TMH3′ ( Fig. 6b ) in the same manner as in the closed C c S state [10] , albeit with the ion further from the Phe380 ring (5.1±0.5 Å on average in the C e S state) than in the closed C c S state [10] (4.6±0.3 Å). Water molecules became inserted between Phe380 and the ion in the simulations of the C e S state ( Fig. 6b ) because the extracellular halves of TMH3′ and TMH6′ are further apart ( Fig. 5d ) than in the closed C c S state ( Table 2 ). These water molecules exchanged readily with bulk waters through the extracellular pathway ( Fig. 7 ). Specifically, ~70 different water molecules came within 3 Å of the Na1′ ion in the outward-facing C e S state and remained for at least 50 ps. Nevertheless, the ion remained coordinated to Thr246 and Thr250 in these simulations ( Fig. 6c ), apparently stabilized by a network of hydrogen bonds formed by, on average, 2.2±0.4 water molecules residing within 3 Å of the Na1′ ion. 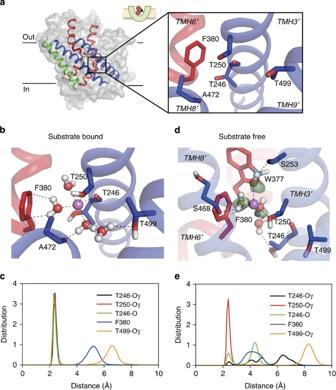Figure 6: The Na1′-binding site in outward-open states of BetP-G153D. (a) The CeS state structure (protomer B) in side view with Na1′ site and adjacent central substrate-binding site in stick representation, coordinating arseno-choline (black, red and purple sticks). The inset shows residues that form the Na1′ site as reported for the closed substrate-bound CcS state. (b–e) The Na1′ site in simulations of the substrate-bound CeS (b,c) and substrate-free Ce(d–e) states: (b,d) example configurations in simulations of the substrate-bound CeS state (b) and the substrate-free Cestate (d). Proteins and ions are presented as in Fig. 6. (c,e) Distances between the Na+ion and protein-binding site atoms (either oxygen, or the center of the phenyl ring in F380) during simulations of the substrate-bound CeS state (c) and the substrate-free Cestate (e). Figure 6: The Na1′-binding site in outward-open states of BetP-G153D. ( a ) The C e S state structure (protomer B) in side view with Na1′ site and adjacent central substrate-binding site in stick representation, coordinating arseno-choline (black, red and purple sticks). The inset shows residues that form the Na1′ site as reported for the closed substrate-bound C c S state. ( b – e ) The Na1′ site in simulations of the substrate-bound C e S ( b , c ) and substrate-free C e ( d – e ) states: ( b,d ) example configurations in simulations of the substrate-bound C e S state ( b ) and the substrate-free C e state ( d ). Proteins and ions are presented as in Fig. 6. ( c , e ) Distances between the Na + ion and protein-binding site atoms (either oxygen, or the center of the phenyl ring in F380) during simulations of the substrate-bound C e S state ( c ) and the substrate-free C e state ( e ). 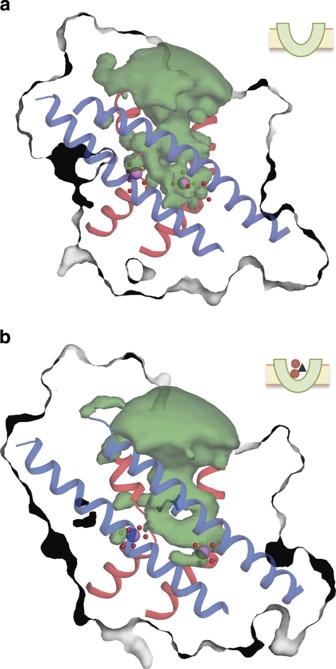Figure 7: Comparison of ion-binding site accessibility and coordination in the substrate-free Ce(a) and substrate-bound CeS (b) states of BetP-G153D observed using molecular dynamics simulations. The green surface indicates the density of water molecules occupying the extracellular pathway (defined as waters within 16 Å of D153) during three 200 ns trajectories. Protein snapshots were taken at 81 and 83 ns of the trajectories of the Ceand CeS states, respectively. BetP protein is shown as a cut-away surface. Sodium ions are shown as violet spheres. Oxygen atoms of water and protein that form the Na2- and Na1′-binding site in the closed CcS state are shown as red spheres. Oxygen atoms in addition to those from the closed-state structure coordinating the ion during molecular simulations of the corresponding state are shown as yellow spheres. Selected helices are shown as cartoons: TMH1′ and its symmetry equivalent TMH6′ (red), and TMH3′ and its symmetry equivalent TMH8′ (blue), with substrate choline shown as sticks. Full size image Figure 7: Comparison of ion-binding site accessibility and coordination in the substrate-free C e (a) and substrate-bound C e S (b) states of BetP-G153D observed using molecular dynamics simulations. The green surface indicates the density of water molecules occupying the extracellular pathway (defined as waters within 16 Å of D153) during three 200 ns trajectories. Protein snapshots were taken at 81 and 83 ns of the trajectories of the C e and C e S states, respectively. BetP protein is shown as a cut-away surface. Sodium ions are shown as violet spheres. Oxygen atoms of water and protein that form the Na2- and Na1′-binding site in the closed C c S state are shown as red spheres. Oxygen atoms in addition to those from the closed-state structure coordinating the ion during molecular simulations of the corresponding state are shown as yellow spheres. Selected helices are shown as cartoons: TMH1′ and its symmetry equivalent TMH6′ (red), and TMH3′ and its symmetry equivalent TMH8′ (blue), with substrate choline shown as sticks. Full size image We also compared the Na1′ site in the C e S state ( Fig. 6a–c ) with that in the C e state ( Fig. 6d,e ), and found a similar situation to that described above for the Na2 site. That is, the sodium ion lacked a typical coordination shell in the C e state, and yet remained coordinated to one or more of the same ligands (the side-chain hydroxyl of Thr250 in this case), with all other ligands then substituted by water molecules ( Fig. 6d ) that were exchanging with the extracellular solution ( Fig. 7 ). These arrangements were formed within 40 ns in three different simulations of the C e state, after initially placing the ion centrally between the binding residues. The altered arrangement of the C e state appears to be attributable to a ~3-Å vertical translocation of TMH9′ relative to TMH3′ ( Fig. 5c ), which separates Thr499 from the other residues in the site ( Figs 5c and 6d ), preventing formation of a stable water bridge that includes two water molecules in the C e S state ( Fig. 6b ) or a single water in the C c S state [10] . In spite of the tenuous and minimal number of direct interactions with the protein, the sodium ion at Na1′ in the C e state formed a stable network of interactions with 3.4±0.5 water molecules ( Figs 6d,e and 7 ). These water molecules in turn formed a network of hydrogen bonds with surrounding groups including, notably, the side chain amine of Trp377 from TMH6′ and the Ser253 hydroxyl from TMH3′, both of which shape the substrate-binding site [2] . The hydrogen bond network also occasionally included the backbone carbonyl of Ala469 or the hydroxyl of Ser468 from TMH8′, which forms the Na2 site ( Fig. 6d ). We reiterate that no positive peak in the Fo-Fc electron-density map at the Na1′ site was observed in the C e S state nor in any of the previously crystallized states of BetP [2] , despite strong evidence that an ion binds to that region, as described above. This lack of a peak might plausibly be a consequence of the dynamic nature of such a well-hydrated ion-binding site, or potentially also of a reduction in occupancy at the Na1′ site in crystals upon dehydration. To date, structures of BetP WT and the choline-transporting mutant BetP-G153D have provided eight distinct conformational states (C eoc , C e Na, C e S, C c S, C ioc S, C i S, C i and C c ) ( Fig. 8 , Supplementary Movies 1–3 ) [2] , [8] , [23] , which after comparison with the crystallized outward- and inward-facing states of Mhp1 and LeuT, revealed similar mechanistic principles but also unique features in each individual system [2] . The choline-transporting BetP-G153D exhibits a higher affinity for Na + than WT protein. This mutant also tends to crystallize in the apo outward-occluded and outward-open states, while the WT crystallizes in either inward or closed states, depending on the concentration of the co-crystallized substrate. Thus, we have now been able to observe substrate in all three main chain conformations, namely C e S, C c S and C i S. This wealth of BetP structures reveals distinct positions of the substrate during its transport trajectory through BetP. While it should be kept in mind that we are comparing structures that have been crystallized with different substrates, we note that the inward-facing C i S state has been observed with both betaine and choline, with nearly identical positions for both trimethyammonium compounds [2] , and therefore the distinct positions observed for substrate in the different states are likely to be physiologically relevant. 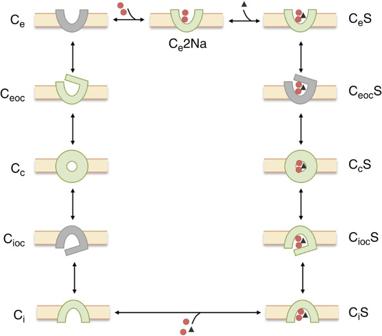Figure 8: The eight conformations of BetP and BetP-G153D determined by X-ray crystallography to date (green): substrate-free outward-open bound to sodium (Ce2Na) (PDB entry 4DOJ); substrate-bound outward-open (CeS) (PDB entry 4LLH, reported here); substrate-bound closed (CcS) (PDB entry 4AIN); substrate-bound inward-occluded (CiocS) (PDB entry 2WIT); substrate-bound inward-open (CiS) (PDB entries 4DOJ/3P03/4AIN/4LLH); substrate-free inward-open (Ci) (PDB entry 4AMR); substrate-free closed (Cc) (PDB entry 4AIN); and substrate-free outward-occluded (Ceoc) (PDB entry 4DOJ). Figure 8: The eight conformations of BetP and BetP-G153D determined by X-ray crystallography to date (green): substrate-free outward-open bound to sodium (C e 2Na) (PDB entry 4DOJ); substrate-bound outward-open (C e S) (PDB entry 4LLH, reported here); substrate-bound closed (C c S) (PDB entry 4AIN); substrate-bound inward-occluded (C ioc S) (PDB entry 2WIT); substrate-bound inward-open (C i S) (PDB entries 4DOJ/3P03/4AIN/4LLH); substrate-free inward-open (C i ) (PDB entry 4AMR); substrate-free closed (C c ) (PDB entry 4AIN); and substrate-free outward-occluded (C eoc ) (PDB entry 4DOJ). Full size image The anomalous scattering demonstrated that arseno-choline is bound to the structure reported here, which allowed a comparison of substrate-free (C e ) and -bound (C e S) outward-open states. MD simulations suggest that sodium is bound, albeit loosely, to both the Na1′ and Na2 sites in both states ( Figs 4 and 6 ), and therefore we reassign the C e structure (monomer B of Protein Data Bank (PDB) entry 4DOJ) to a C e 2Na state ( Fig. 8 ). The observation that an ion remains coordinated at a solvent-accessible Na2 site in the substrate-free C e 2Na state mirrors observations for an outward-open structure of another LeuT-fold transporter, Mhp1 (ref. 6 ). In both transporters, binding of substrate and formation of the C e S state leads to occlusion of the Na2 site from the extracellular solution ( Fig. 7 ) [6] . Our simulations also suggest a concomitant increase in stability of the ion–protein interactions at the Na2 site in the C e S state compared with the C e 2Na state ( Fig. 4 ). These changes reflect a number of small helix reorganizations around the site that improve the Na2 coordination in the C e S state ( Fig. 5b ), rendering it very similar to that in the C c S state ( Table 2 ) [10] . In the case of the Na1′ site, by contrast, the ion is accessible to water in both the C e 2Na and C e S states ( Fig. 7 ). However, similar to Na2, the Na1′ site exhibits significantly fewer stable protein–ion interactions in the C e 2Na state compared with the substrate-bound form (C e S, Fig. 6 ) or the closed C c S state [10] , due to the shift in TMH9′ ( Fig. 5C ). Complete closure of the periplasmic pathway in the transition between the two holo forms (C e S to C c S) involves further contraction of TMH3′ and TMH9′ towards TMH8′ ( Fig. 5d ), which brings the ion ~0.5 Å closer to F380 ( Fig. 6 cf. (ref. 10 )). Meta-stable ion-binding sites, such as those seen here for the C e 2Na state, that are proximal to, and involve a number of ligands from, the main binding sites, may be useful because they enhance the local ion concentration. Indeed, solvated, meta-stable sites appear to be a common theme for ion-coupled transporters, and have been identified during MD simulations and free-energy calculations of vSGLT [20] , [21] and Mhp1 [24] , as well as LeuT [25] . The important role of individual water molecules binding sodium within transporter proteins is underlined by the ion-water coordination observed in a recent structure of Drosophila melanogaster dopamine transporter (dDAT) [26] , as well as in c-subunits of ATP-synthase rotor rings [27] . Together, these results suggest a sequential Na + /substrate-binding process in which ions are loosely associated with partially formed, partially hydrated Na1′ and Na2 sites in the outward-open state, in the absence of substrate. Studies of other LeuT homologues indicate distinct roles for the two cations in transport [28] , [29] , [30] , [31] , [32] and, in terms of binding order, the most likely scenario appears to be that Na2 would bind before Na1 [28] . Indeed, spectroscopic and computational evidence that sodium shifts the equilibrium of LeuT towards opening of the central binding site to the periplasm [11] , [12] , [24] ; this, combined with the fact that the Na2 site is conserved among sodium-coupled transporters, suggests that Na2 is required for the conformational change. A similar mechanism may be adopted by BetP since the Na2 site residues are closer together in the outward-open states than in the inward-open states ( Table 2 ). The finding that both ions bind to the empty transporter before substrate is consistent with electrophysiological studies of human Na + -coupled glucose symporter (hSGLT1), a homologue of vSGLT [30] . In the case of BetP and Mhp1, one effect of substrate binding is to occlude the Na2 site, which should reduce the probability of ion unbinding [6] , [24] . Complete closure to form the C c S state then involves optimization of the binding interactions, at which point the energy gained by binding is maximal. By analogy with enzymatic mechanisms, this closed state is therefore a transition state, in line with the induced transition fit model proposed by Klingenberg [33] . However, further analysis of BetP will be required to further validate this hypothesis. For example, in future work it would be of interest to follow the approach of Loo et al. [30] , and to compute the potential of mean force of the ions along their pathway into the binding sites in BetP to predict whether there is a significant barrier to formation of these assumed states. In conclusion, results from a combination of structural studies and molecular simulations reveal for the first time for a secondary transporter how binding of coupling ions may involve progressive dehydration and concurrent coordination by protein residues. Studies of subsequent steps in the cycle will be required to address the question of whether the binding steps alone, or other later events, determine the strict ion-substrate coupling in BetP. Synthesis of arseno-choline Arseno-choline was obtained [34] by heating trimethylarsine with bromo-ethanol, followed by re-crystallization from methanol/acetone; the purity (>99.5%) of the compounds was established by NMR spectroscopy and HPLC/mass spectrometry (MS) (inductively coupled plasma MS and electrospray MS). Cell culturing and protein purification Cell culture and protein preparation methods have been described previously [23] . Briefly, E. coli DH5αmcr [35] were used for the heterologous expression of strep-betP. Cells were grown at 37 °C in LB medium supplemented with carbenicillin (50 μg ml −1 ) and induction was initiated with anhydrotetracycline (200 μg l −1 ). Cells were harvested at 4 °C by centrifugation and resuspended in buffer containing 100 mM Tris–HCl (pH 8.0) and protease inhibitor Pefabloc 0.24 mg ml −1 . Membranes were isolated from disrupted cells and solubilized with 1% β-dodecyl-maltoside (DDM) when purified protein was subsequently crystallized or reconstituted. The protein was then loaded on a StrepII-Tactin macroprep column, washed with 50 mM Tris–HCl (pH 7.5), 500 mM NaCl, 8.6% glycerol, 0.1% DDM and eluted with 5 mM desthiobiotin, 50 mM Tris-HCl (pH 7.5), 200 mM NaCl, 8.7% glycerol and 0.6% Cymal-5, if used for crystallization, or 0.1% DDM if used for reconstitution. Before crystallization the protein was loaded onto a Superose 6 (GE Healthcare) size-exclusion column equilibrated with 20 mM Tris–HCl (pH 7.5), 200 mM NaCl and 0.6% Cymal-5. This purified protein was concentrated at 4 °C to ~10 mg ml −1 at 3,000 g in a Vivaspin tube (Vivascience) with a 100-k-molecular-weight cutoff, and incubated for 16 h at 4 °C with either 8 mM arseno-choline or 1 mM arseno-betaine. Site-directed mutagenesis Site-directed mutagenesis of the pASK-IBA5betP20 and pASK IBA7betPΔN29/E44E45E46/AAA23 plasmids were performed using the QuickChangeTM kit (Stratagene), Pfu Turbo DNA polymerase and specific Oligonucleotides. The mutations were verified by nucleotide sequencing. The fully functional mutant BetP(ΔN29/E44E45E46/AAA/G153D) was used for crystallization purposes yielding in improved diffraction power and isotropy of the crystals. Crystallization and structure determination BetP-ΔN29/E44E45E46/AAA/G153D was co-crystallized with 8 mM arseno-choline at 18 °C by vapour diffusion in hanging drops of 1 μl protein solution with 1 μl of 100 mM Na-tri-citrate (pH 5.3–5.6), 300 mM NaCl or RbCl and 17–24% PEG 400 as reservoir solution. Crystals of BetP-ΔN29/EEE44/45/46AAA/G153D diffracted to 2.9 Å, and data were collected on the beamline PXII at the Swiss Light Source (Swiss Light Source at the Paul Scherrer Institut, Villigen, Switzerland). Data were collected at the K edge for arsenic, using a wavelength of ~1.043 Å. Data were processed using the XDS package [36] and the anisotropy was corrected on the UCLA Diffraction Anisotropy Server ( http://services.mbi.ucla.edu/anisoscale/ ) [37] . Structure was determined by molecular replacement with BetP (PDB entry 4DOJ) as search model using PHASER [38] and refinement was performed using PHENIX [39] combined with manual rebuilding in COOT [40] . Protein reconstitution into liposomes Functional reconstitution of BetP-G153 was performed as described [41] . Briefly, liposomes (20 mg phospholipid ml −1 ) from E. coli polar lipids (Avanti polar lipids) were prepared by extrusion through polycarbonate filters (100 nm pore size) and diluted 1:4 in buffer (250 mM KPi pH 7.5). After saturation with Triton X-100, the liposomes were mixed with purified protein at a lipid/protein ratio of 10:1 (w/w). BioBeads at ratios (w/w) of 5 (BioBeads/Triton X-100) and 10 (BioBeads/DDM) were added to remove detergent. Finally, the proteoliposomes were centrifuged and washed before being frozen in liquid nitrogen and stored at −80 °C. Tryptophan fluorescence-binding assay Binding assays were performed with 100 μg ml −1 of purified BetP-G153D in proteoliposomes [41] . Choline and arseno-choline concentrations ranged from 0.1 to 16 mM for measurements at 100 mM NaCl and pH 7.5. Choline concentrations ranged from 0.8 to 30 mM at pH 5.5 and 0.8 to 100 mM at pH 7.5 in absence of NaCl. Tryptophan fluorescence emission between 315 and 370 nm was recorded on a Hitachi F-4500 fluorescence spectrophotometer and averaged over eight readings, with the excitation wavelength set to 295 nm and a slit width of 2.5 or 5.0 nm for excitation or emission, respectively. The mean value and s.d. at the 340-nm emission maximum was plotted for each substrate concentration. Binding constants were derived by fitting with the program GraphPad Prism version 5.0c for Mac OS X, GraphPad Software [42] . SSM-based electrophysiology SSM-based electrophysiology was performed as described [10] , [43] , [44] using 40 μl of proteoliposomes at a protein concentration of 1 mg ml −1 . Briefly, experiments were carried out at room temperature (22 °C). The solution-exchange protocol consisted of four phases with a total duration 4.8 s. (i) non-activating solution (2.5 s), (ii) activating solution (0.8 s), (iii) non-activating solution (0.5 s) and (iv) resting solution (1.0 s). The resting solution was composed of 250 mM KPi buffer (7.5). Non-activating and activating solution also contained 250 mM KPi buffer (pH 7.5). The osmolality of non-activating and activating solution was kept constant. Activation by choline or arseno-choline was performed using a non-activating solution with x μM glycine plus 500 mM NaCl and an activating solution with corresponding x μM choline or arseno-choline plus 500 mM NaCl. Thereby an osmolar gradient was established when switching from the resting to the non-activating solution at the start of the experiment. Note that during the final experiments (several minutes) the cuvette contained resting solution to ensure low osmolar conditions in the proteoliposomes. Transient currents were recorded at the concentration jumps taking place from non-activating to activating buffers. The current amplifier was set to a gain of 10 9 –10 10 V A −1 , and low-pass filtering was a 300–1,000 Hz. Transport assays Uptake of [ 14 C]-betaine in E. coli cells was performed as described [45] . E. coli MKH13 cells expressing a particular strep-betP mutant were cultivated at 37 °C in LB medium containing carbenicillin (50 μg ml −1 ) and induced at an OD 600 of 0.5 by adding anhydrotetracycline (200 μg l −1 ). After 2 h the cells were harvested and washed in buffer containing 25 mM KPi buffer (pH 7.5) and then were resuspended in the same buffer containing 20 mM glucose. For uptake measurements the external osmolality was adjusted with KCl at a constant value of 800 mOsmol kg −1 . Sodium titration was performed by adjusting the NaCl concentration in the buffer. Cells were incubated for 3 min at 37 °C before the addition of 250 μM [ 14 C]-betaine. Betaine uptake was measured at various time intervals, after cell samples were passed through glass fibre filters (APFF02500; Millipore) and were washed twice with 2.5 ml of 0.6 M KPi buffer. The radioactivity retained on the filters was quantified by liquid scintillation counting. MD simulations MD simulations were carried for monomers taken from two different crystallographic structures: (1) monomers A and B of the structure presented here (PDB 4LLH), which are both in outward-open substrate-bound (C e S) states; and (2) monomer B of PDB entry 4DOJ, which is in an outward-open apo (C e ) state. Protonation states were assigned according to calculations performed on the X-ray structures using MCCE2.0 [46] . Specifically, residues His188, His192, His445, His482 and His570 were protonated at their Nɛ atom while His176, His176 and His573 were protonated at their Nδ atoms. On the basis of the same calculations, Glu161 was assumed to be neutral, while Asp153 was charged. The likely location of buried water molecules was identified using DOWSER [47] . The protein was inserted into a 50:50 diastereoisomeric mixture of 219 palmitoyl oleoyl phosphatidyl-glycerol (POPG) lipid molecules, hydrated with salt water. Specifically, monomers A and B of the C e S state were solvated by 15,140 and 15,149 water molecules, plus 245 and 254 sodium ions, respectively, and the C e structure was solvated by 15,126 water molecules and 253 sodium ions. All three systems also contain 27 chloride ions to neutralize any net charge and to maintain an ~0.15 M salt concentration. The final systems were ~91 × 91 × 96 Å in size. In the C e S structures, a substrate choline molecule and an ion at Na2 were placed according to positive peaks observed in the F o −F c difference-density map, whereas the sodium at Na1′ was placed equidistant between the hydroxyl oxygen atoms of T246 and T250 and the center of the F380 phenyl ring. A water molecule was placed adjacent to the Na1′ so as to indirectly coordinate T499 (ref. 10 ). In the C e structure, sodium ions were placed based on superposition of the simulated C c S structure (monomer B of 4AIN). The complete monomer-bilayer system was set up using GRIFFIN [48] . Briefly, GRIFFIN was first used to carve out lipid and water molecules from the equivalent volume of the protein. Subsequently, a three-step optimization was performed, with each step 50 ps long and with external forces of 1.0, 2.0, then 3.0 kcal mol −1 Å 2 or 1.0, 1.5 then 2.0 kcal mol −1 Å 2 used for the C e or C e S structures, respectively. After 1,000 steps of conjugate gradients energy minimization, 20 ns of MD simulation was carried out in which all non-hydrogen atoms of the protein, ligand and bound sodium ions were constrained to their initial positions using springs with progressively smaller force constants, starting at 15 kcal mol −1 Å 2 . During the equilibration of the C e S state, distance constraints were applied between choline and the tryptophan box (W373, W374 and W377) as well as with D153, in order to maintain the substrate orientation and position as in the C e S X-ray structures. Similarly, the distances between sodium ions and their coordinating residues (T246, T250 and F380 for Na1 and A147, M150, F464, T467 and S468 for Na2) were constrained. Analysis was carried out every ps of unconstrained simulations, each 200 ns (for C e S) or 100 ns (for C e ) in length. All MD simulations were performed using NAMD [49] . Periodic boundary conditions were used. A real-space cutoff of 12 Å was used for both van der Waals and long-range electrostatics; the distance at which the switching function began to take effect was 10 Å. The time step was 2 fs. The SHAKE algorithm [50] was used to fix all bond lengths. Constant temperature (310 K) was set with a Langevin thermostat [51] , with a coupling coefficient of 0.2 ps −1 . A Nosé–Hoover Langevin barostat [52] was used to apply constant pressure normal to the membrane plane, with an oscillation period of 200 fs and the damping time scale set to 50 fs. The surface area in the membrane plane was kept constant. The all-atom CHARMM27 force field was used for protein [53] , [54] and ions [55] , and TIP3P was used for water molecules [56] . Force field parameters for POPG were kindly provided by H. Jang (National Cancer Institute, Frederick, MD) [57] . The parameters for choline were taken from the CHARMM general force field (CGenFF) topology and parameter files [58] . The MD trajectories were analysed with CHARMM and visual MD [59] . Accession codes. Coordinates and structure factors for the outward-open state of BetP have been deposited in the RCSB Protein Data Bank under accession code 4LLH . How to cite this article: Perez, C. et al. Substrate-bound outward-open state of the betaine transporter BetP provides insights into Na + coupling. Nat. Commun. 5:4231 doi: 10.1038/ncomms5231 (2014).